Active microrheology and simultaneous visualization of sheared phospholipid monolayers Two-dimensional films of surface-active agents—from phospholipids and proteins to nanoparticles and colloids—stabilize fluid interfaces, which are essential to the science, technology and engineering of everyday life. The 2D nature of interfaces present unique challenges and opportunities: coupling between the 2D films and the bulk fluids complicates the measurement of surface dynamic properties, but allows the interfacial microstructure to be directly visualized during deformation. Here we present a novel technique that combines active microrheology with fluorescence microscopy to visualize fluid interfaces as they deform under applied stress, allowing structure and rheology to be correlated on the micron-scale in monolayer films. We show that even simple, single-component lipid monolayers can exhibit viscoelasticity, history dependence, a yield stress and hours-long time scales for elastic recoil and aging. Simultaneous visualization of the monolayer under stress shows that the rich dynamical response results from the cooperative dynamics and deformation of liquid-crystalline domains and their boundaries. Fluid interfaces are ubiquitous in industry, technology and life [1] . Interfaces separate and organize biological systems [2] , [3] , from organelles to cells to organs, and enable gas exchange in respiration [4] . High-interface foams and emulsions find wide use in industry, food and personal care products [5] : emulsified oil droplets give both taste and texture to a fine espresso. Surfactants, including traditional amphiphilic fatty acids and phospholipids [2] , [3] , [4] , [6] , [7] and non-traditional surfactants, such as colloids [8] , [9] , block copolymers [10] and nanoparticles [11] , lower the free energy of interfaces and introduce a kinetic barrier to coalescence, thereby stabilizing these high-interface systems [6] by creating novel microstructures and phases. The static properties of interfaces have long been studied: Langmuir isotherms relate the surface tension, γ , (or the surface pressure Π= γ (0)– γ (Γ)), to the surface concentration, Γ, of surfactant [12] , [13] . However, the dynamic properties of interfaces—how monolayers and bilayers respond to applied forces—can be equally important, albeit less well known. The dynamic response is more challenging to study, as the bulk material generally swamps the interfacial viscoelastic response in a conventional rheometer. Probes moving within the interface feel drag from both the interface and the bulk fluid. To maximize sensitivity to the interfacial properties, the Boussinesq number, must be large [1] , [14] , [15] , [16] , [17] . Here η s and η are the viscosities of the interface and the bulk, and P c and A c are the contact perimeter and wetted surface area of the probe. Bo establishes a practical lower limit, η s > ηA c / P c , that can be measured with a given probe. High-aspect ratio probes such as knife-edges [1] or magnetic needles [14] , [15] , [16] , [17] maximize sensitivity, and even larger P c / A c ratios can be achieved with micron-scale colloidal spheres [18] , [19] or ferromagnetic nanorods [16] , [20] . Here we describe a new active microrheology technique sensitive to the surface viscoelasticity of a wide range of interfaces. Using photolithography, we make micron-scale, ferromagnetic 'microbuttons', whose surface chemistry is tuned to render them amphiphilic ( Fig. 1 ). A known torque is applied by electromagnets to rotate a microbutton at the interface, and the 'buttonholes' are tracked to record the angular displacement as a function of time. The result is a micron-scale, two-dimensional (2D) Couette rheometer with P c / A c ∼ 1/ R ∼ 1/(10 μm) that can measure surface viscosities of order η s ∼ O(10 −8 ) N s m −1 (| Bo |>1), and can simultaneously follow the evolution of the interfacial microstructure with fluorescence microscopy. Our work builds on related, larger-scale techniques [21] , [22] , adding not only dramatically enhanced sensitivity but also simultaneous visualization [23] . Such direct correlation is almost impossible in traditional, three-dimensional (3D) rheology [24] , [25] . 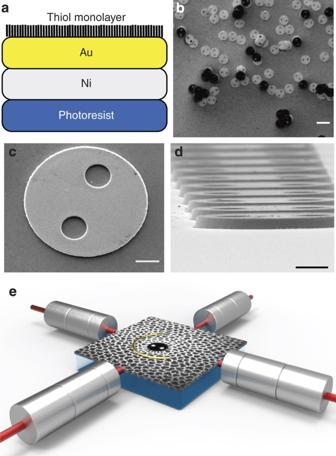Figure 1: Ferromagnetic 'microbutton' probes. (a) Ferromagnetic Janus (two-faced) 'microbutton' probes are fabricated photolithographically from SU-8 photoresist, evaporatively coated with ferromagnetic (nickel) and gold layers, and made amphiphilic by depositing alkane-thiol or fluorocarbon-thiol monolayers on the gold34. (b–d) Scanning electron microscopy images showing (b) the Janus character of the microbuttons (photoresist appears dark, thiol-gold appears light; scale bar, 20 μm). Higher-magnification images of (c) a microbutton (20 μm diameter) showing buttonholes (5 μm diameter) and (d) an as-fabricated array showing a uniform 1 μm thickness (scale bar, 5 μm). (e) Active, interfacial microrheometry: a ferromagnetic microbutton is placed within a surfactant monolayer on a water/air interface. Computer-controlled electromagnets exert a defined torque (stress) on the microbutton, whose rotation (strain) is recorded with bright-field microscopy, along with simultaneous fluorescence video microscopy of the monolayer. Figure 1: Ferromagnetic 'microbutton' probes. ( a ) Ferromagnetic Janus (two-faced) 'microbutton' probes are fabricated photolithographically from SU-8 photoresist, evaporatively coated with ferromagnetic (nickel) and gold layers, and made amphiphilic by depositing alkane-thiol or fluorocarbon-thiol monolayers on the gold [34] . ( b – d ) Scanning electron microscopy images showing ( b ) the Janus character of the microbuttons (photoresist appears dark, thiol-gold appears light; scale bar, 20 μm). Higher-magnification images of ( c ) a microbutton (20 μm diameter) showing buttonholes (5 μm diameter) and ( d ) an as-fabricated array showing a uniform 1 μm thickness (scale bar, 5 μm). ( e ) Active, interfacial microrheometry: a ferromagnetic microbutton is placed within a surfactant monolayer on a water/air interface. Computer-controlled electromagnets exert a defined torque (stress) on the microbutton, whose rotation (strain) is recorded with bright-field microscopy, along with simultaneous fluorescence video microscopy of the monolayer. Full size image Frequency-dependent linear viscoelasticity of liquid-condensed dipalmitoylphosphatidylcholine Here we show that the monolayer dynamics of even a single-component monolayer of dipalmitoylphosphatidylcholine (DPPC), one of the primary lipids in lung surfactant [5] , [7] and ubiquitous in cell membranes, can be far richer than ever expected. DPPC monolayers exhibit a disordered liquid-expanded (LE) phase at low surface pressures that transforms into a liquid-condensed (LC) phase with long-range orientational and short-range positional order (hexatic) at Π=7 mN m −1 at 20 °C ( Fig. 1 ) [2] , [3] , [13] , [26] , [27] . All experiments are performed at Π=9±1 mN m −1 in the LC phase, just above the coexistence plateau. A small-amplitude, oscillatory magnetic field, , applied perpendicular to the magnetic moment, , of a microbutton suspended at the interface ( Fig. 1 ), exerts an oscillatory torque that drives a small oscillatory rotation . Measuring the buttonhole orientation along with the applied torque determines the probe's rotational resistance . When Bo ≫ 1, the real and imaginary parts of ζ ( ω ) are proportional to the surface elastic and viscous shear moduli, G ′ s ( ω ) and G ′′ s ( ω )= ωη s ( ω ), respectively. Much to our surprise, the DPPC monolayer had a primarily elastic response (G′ s ∼ 150 nN m −1 ) down to 0.1 Hz, indicating that the monolayer stored elastic energy, without appreciable relaxation, over 10-s time scales ( Fig. 2a–c ). Above 4 Hz, however, G ′ s ( ω ) and G ′′ s ( ω ) crossed, and the monolayer response was primarily viscous ( η s ∼ 70 nN s m −1 ) ( Supplementary Movie 1 ). 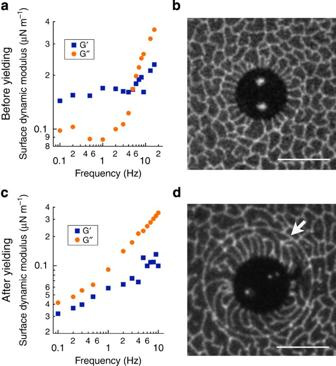Figure 2: History-dependent linear viscoelasticity. (a) Linear viscoelasticity of as-prepared liquid-condensed dipalmitoylphosphatidylcholine (LC-DPPC) monolayers at air/water interfaces (Π=9±1 mN m−1). Surface shear moduli indicate a dominant low-frequency elastic response,G′s(ω)>G′′s(ω) down to 0.1 Hz, crossing over to a primarily viscous response,G′′s(ω)>G′s(ω) above 5 Hz. (b) Direct visualization of the DPPC monolayer reveals the elastic response to result from a network of interlocked LC domains that cannot deform without deforming neighbouring domains. (c) After forcing a large-amplitude microbutton rotation, LC-DPPC appears viscousG′′s(ω)>G′s(ω) at all frequencies. (d) Visualization reveals the creation of a 'slip line' (white arrow) within the monolayer, which enables non-cooperative deformation under shear (scale bar, 20 μm). Figure 2: History-dependent linear viscoelasticity. ( a ) Linear viscoelasticity of as-prepared liquid-condensed dipalmitoylphosphatidylcholine (LC-DPPC) monolayers at air/water interfaces (Π=9±1 mN m −1 ). Surface shear moduli indicate a dominant low-frequency elastic response, G ′ s ( ω )> G ′′ s ( ω ) down to 0.1 Hz, crossing over to a primarily viscous response, G ′′ s ( ω )> G ′ s ( ω ) above 5 Hz. ( b ) Direct visualization of the DPPC monolayer reveals the elastic response to result from a network of interlocked LC domains that cannot deform without deforming neighbouring domains. ( c ) After forcing a large-amplitude microbutton rotation, LC-DPPC appears viscous G ′′ s ( ω )> G ′ s ( ω ) at all frequencies. ( d ) Visualization reveals the creation of a 'slip line' (white arrow) within the monolayer, which enables non-cooperative deformation under shear (scale bar, 20 μm). Full size image History-dependent rheology of DPPC Forcing a few large-amplitude (180°) rotations, however, changed the measured response dramatically ( Fig. 2d–f ). The DPPC monolayer exhibited a viscous (albeit frequency-thinning) response at all frequencies measured, without the elastic storage seen in a 'freshly prepared' monolayer. This dramatic history-dependence highlights the care required in interpreting dynamic measurements of monolayers. Our ability to visualize the monolayer while deforming it allowed us to unambiguously identify the microstructure changes responsible for this unusual behaviour. The bright lines (high fluorescent dye concentration) in Figure 2c and Supplementary Movie 1 show the boundaries of the irregularly shaped, interlocking ∼ 10 μm LC domains [2] , which cannot slide past each other without deforming. DPPC monolayers in the LC phase respond to a weak applied stress with small elastic deformations of the domains, rather than rearrangement of the domains or the domain boundaries [24] . Large-amplitude deformations, however, drive the monolayer out of its equilibrium microstructure ( Fig. 2f and Supplementary Movie 2 ). The domains deform enough that the boundary forms a continuous, almost circular slip line that effectively fractures the material. The microbutton and domains within the slip line rotate freely, with minimal deformation of the domains inside or outside of the slip line, eliminating the elastic response ( Fig. 2d,e ). Ageing and healing of a single slip line On returning the microbutton to its original orientation and removing the driving torque, the circular slip line roughens ( Fig. 3 ), the smoothed grains heal to their interpenetrating configuration (compare Fig. 3a, e ), and the original viscoelastic response ( Fig. 3f ) is recovered. When the slip line is formed ( Fig. 3b ), both G ′ s and G ′′ s drop 20- to 100-fold ( Fig. 3f ), and the monolayer appears primarily viscous ( G ′′ s > G ′ s ). However, after shear stops, both G ′ s and G ′′ s increase with time: the elastic response is recovered ( G ′ s > G ′′ s ) after 40 s, when the domain structures again interpenetrate ( Fig. 3c ). Even the detailed features of the grain boundaries and domains are largely restored after 150 s ( Fig. 3e ). 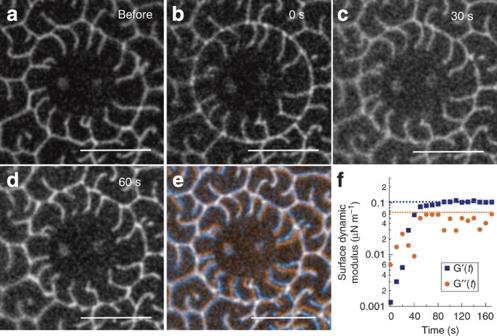Figure 3: A fractured monolayer heals. (a) Initially, domains around a microbutton form a rough boundary with neighbouring domains. (b) Forcing a large-amplitude rotation smoothes the boundary to a nearly circular slip line, reduces the linear viscoelastic response 20- to 100-fold (f) and eliminates the elastic response. (c, d) Line tension progressively roughens the slip line, with an accompanying increase in surface shear modulus (f). (e) Overlaying initial (red) and final (blue,t=60 s) images reveals the domain structure has healed almost completely, highlighting a remarkably persistent memory (scale bar, 20 μm). Figure 3: A fractured monolayer heals. ( a ) Initially, domains around a microbutton form a rough boundary with neighbouring domains. ( b ) Forcing a large-amplitude rotation smoothes the boundary to a nearly circular slip line, reduces the linear viscoelastic response 20- to 100-fold ( f ) and eliminates the elastic response. ( c, d ) Line tension progressively roughens the slip line, with an accompanying increase in surface shear modulus ( f ). ( e ) Overlaying initial (red) and final (blue, t =60 s) images reveals the domain structure has healed almost completely, highlighting a remarkably persistent memory (scale bar, 20 μm). Full size image Surface yield stress measurements from steady rotation Significant domain deformation should require a stress of order G ′ s as well: concentrated emulsions yield at applied stresses of ∼ G ′/10 (refs 5 , 28 , 29 ). Monolayers respond to a steady torque ( Fig. 4 and Supplementary Movie 3 ) by establishing two distinct regions: an outer region in which the interface does not flow, and an inner region that appears largely structure-free and freely flowing. The boundary radius, R Y , between the two is determined by the surface yield stress, τ s Y : the interface flows for r < R Y where τ s > τ s Y , but deforms elastically for r > R Y where τ s < τ s Y . An interfacial torque balance relates applied torque to surface shear as T app =2 πR Y 2 τ s Y . 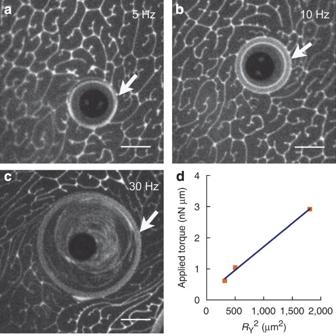Figure 4: Yield stress measurement. Steady rotation at 5 Hz (a), 10 Hz (b), and 30 Hz (c) divides the monolayer into two regions: an inner region that flows with the microbutton, deforms continuously and appears domain-free; and an outer region with domains that does not deform significantly. The radiusRYof the yielded region (white arrows) is set by the surface yield stress,τsY. A torque balance givesTapp=2πRY2τsY, consistent with (d); the slope givesτsY∼10−2μN m−1,∼G′s(ω)/10 (Fig. 2) as expected by analogy with three-dimensional emulsions5,28,29(scale bar, 20 μm). Figure 4d shows that T app increases linearly with R Y 2 , whose slope gives a surface yield stress τ s Y ∼ 0.01 μN m −1 of order G ′ s /10, as expected [5] , [28] , [29] . Figure 4: Yield stress measurement. Steady rotation at 5 Hz ( a ), 10 Hz ( b ), and 30 Hz ( c ) divides the monolayer into two regions: an inner region that flows with the microbutton, deforms continuously and appears domain-free; and an outer region with domains that does not deform significantly. The radius R Y of the yielded region (white arrows) is set by the surface yield stress, τ s Y . A torque balance gives T app =2 πR Y 2 τ s Y , consistent with ( d ); the slope gives τ s Y ∼ 10 −2 μN m −1 , ∼ G ′ s ( ω )/10 ( Fig. 2 ) as expected by analogy with three-dimensional emulsions [5] , [28] , [29] (scale bar, 20 μm). Full size image Hours-long viscoelastic recovery after steady shear The division into flowing (yielded) and elastic regions is reminiscent of many other yield-stress materials [30] whose yield stress results from an interlocking or system-spanning elastic network. Forcing such materials to flow destroys this structure, which gradually heals when the imposed shear is removed. The LC-DPPC monolayer, however, did not age in a straightforward manner once the driving torque was removed. Instead, to our great surprise, steadily sheared monolayers immediately begin to recoil and 'unwind' for minutes to even hours ( Fig. 5 and Supplementary Movie 4 ). 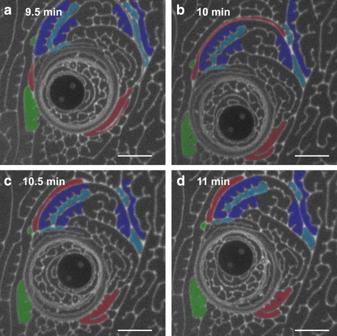Figure 5: Evolution of the yielded region following 5 min of 60 Hz microbutton rotation. Although the yielded region had appeared to be largely domain-free (Fig. 4), discrete but highly deformed LC domains have maintained their identity and liquid-crystalline orientational order. (a–d) After the stress has been relieved, line tension pulls domains (red) from imperceptibly thin, extended structures (a) to more energetically favourable compact structures (d). Domains exchange neighbours by relative sliding (green), and topological 'T1' transitions, wherein domains that are initially North–South neighbours (light-blue) make way for East–West neighbours (dark-blue) as during the coarsening of foams and emulsions5(scale bar, 20 μm). Figure 5: Evolution of the yielded region following 5 min of 60 Hz microbutton rotation. Although the yielded region had appeared to be largely domain-free ( Fig. 4 ), discrete but highly deformed LC domains have maintained their identity and liquid-crystalline orientational order. ( a – d ) After the stress has been relieved, line tension pulls domains (red) from imperceptibly thin, extended structures ( a ) to more energetically favourable compact structures ( d ). Domains exchange neighbours by relative sliding (green), and topological 'T1' transitions, wherein domains that are initially North–South neighbours (light-blue) make way for East–West neighbours (dark-blue) as during the coarsening of foams and emulsions [5] (scale bar, 20 μm). Full size image The low-frequency, linear elastic response, followed by flow at larger strains also arises in concentrated 3D emulsions, which cannot rearrange unless the applied stress is sufficiently strong to significantly deform the tightly packed droplets [5] . Emulsions deform elastically until a critical yield stress is applied, above which they flow: mayonnaise sits like a solid under gravity, but may be easily spread with a knife. In 3D emulsions, elastic energy is stored in droplet interfaces, giving G ′ s ∼ γ / R d for droplets of size R d and surface tension γ [5] , [28] , [29] . Extending this analogy to 2D emulsions suggests the measured surface elastic modulus G ′ s ∼ λ / R d ∼ 0.15 μN m −1 is set by the line tension of the domain boundaries, λ , and the size, R d ∼ 10 μm, of the LC domains. The resulting line tension, λ ∼ G ′ s R d ∼ 1 pN, is in good agreement with measured values for phospholipid and fatty acid monolayers [31] , and is consistent with a simple molecular argument: The attractive energy between molecules in a condensed liquid phase must be of order k B T, so the energy cost of moving from an ordered to disordered liquid should be ∼ k B T per molecule. Given a line density ∼ 1 molecule per nm, one expects a line energy λ ∼ k B T nm −1 ∼ pN. Figure 5 highlights the recovery of a monolayer that had been sheared at 60 Hz for 5 min, then allowed to relax. Domains slip relative to one another (green) or neighbouring pairs can swap (adjacent light-blue domains make way for dark-blue domains to be neighbours) through topological transitions reminiscent of T1 events in foams and concentrated emulsions [5] . Unlike 3D emulsions, however, highly stretched domains (red) evolve from imperceptibly thin crescents to increasingly compact structures. Such extended shapes may at first seem surprising: stretched droplets in 3D emulsions break into smaller droplets because of the Plateau–Rayleigh (capillary) instability. The absence of out-of-plane curvature in 2D, however, makes the stretched domains inherently 'stable' [32] , [33] . 2D domains can thus stretch without breaking, maintaining their integrity while slipping past each other, until they may eventually become so thin that non-hydrodynamic forces cause their rupture. Once stress is removed, the line tension of the still-continuous boundaries acts to pull the domains back into more energetically favourable compact configurations. The dynamics of steadily sheared LC monolayers and their subsequent relaxation are generally quite complicated. If the topology of the domain structure were rigorously preserved (for example, domains could not slip, rearrange or break), the recovery would be complete and elastic, as indeed occurs for small applied rotations ( Fig. 6 ). The relatively inviscid grain boundaries, however, allow stretched grains to slide along the slip lines that form within the yielding monolayer, swapping neighbours rather than deforming further. Nonetheless, the disc drives shear deformations that continually stretch and arrange domains in a 'wound' manner, even as they respond by slipping, rearranging and perhaps even breaking. Once shear is removed, line tension clearly drives the monolayer to recoil, whether the domains retain their topology or not. 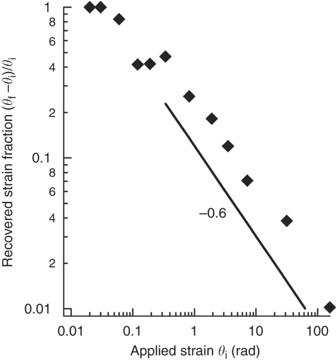Figure 6: Fraction of strain recovered as microbutton 'unwinds' after torque is removed. Recovered strain fraction (θf−θi)/θiis measured as a function of initial, applied strainθi. The recovered strain fraction shows a power-law behaviour, decaying with initial strain to the −0.6 power. Topological rearragements (for example, domain slipping and neighbour swapping) and general viscoelastic deformations irreversibly lose elastic energy that would otherwise be stored while 'winding'. Topological changes and viscous losses thus generally give rise to a viscoelastic (partial) recovery: Figure 6 reveals the recovered (unwound) fraction to decay with applied strain by an approximate power-law −0.6. Figure 6: Fraction of strain recovered as microbutton 'unwinds' after torque is removed. Recovered strain fraction ( θ f −θ i )/ θ i is measured as a function of initial, applied strain θ i . The recovered strain fraction shows a power-law behaviour, decaying with initial strain to the −0.6 power. Topological rearragements (for example, domain slipping and neighbour swapping) and general viscoelastic deformations irreversibly lose elastic energy that would otherwise be stored while 'winding'. Full size image Our measurements and observations lead us to argue that LC-DPPC monolayers—and likely grainy LC monolayers in general—behave like high-internal phase emulsions, but with novel 2D features. Line tension drives domains towards lower-energy shapes against an inhomogeneous viscous resistance: viscous grains are separated by relatively inviscid boundaries. Under small strains, the interpenetrating LC grains deform only slightly, but cooperatively, to give a viscoelastic response ( Fig. 2 ). Large-amplitude oscillatory strains smooth the interpenetrations to form slip lines, along which localized, non-cooperative deformations occur with little resistance. If domains have not rearranged, however, 'smoothed' slip lines roughen to recover their initial (equilibrium) structure ( Fig. 3 ). Monolayers fully yield under steady shear, forming extended (yet continuous) domains that continually slip past one another along multiple slip lines. Line tension pulls extended grains back into more compact shapes against the high LC viscosity, while grains rearrange and slide relative to one another along local slip lines. By visualizing the structure of an interface while it is being deformed, our new technique provides an unprecedented ability to correlate structural deformations with rheological response. More generally, our technique can interrogate the dynamical response of a wide variety of fluid/fluid interfaces, of scientific, biological, industrial and technological relevance. For example, lipids, proteins and fatty acids can be added to systematically construct model monolayers of biological relevance, such as the lung surfactant monolayer [4] , [7] , [17] . Fabrication of amphiphilic ferromagnetic microbuttons We use photolithography to fabricate micron-scale, ferromagnetic, amphiphilic 'microbutton' probes, as described in detail elsewhere [34] . Briefly, a 4 inch diameter silicon wafer is cleaned with piranha solution, and a 200 nm sacrificial layer (Omnicoat, Microchem) is spin-coated onto the wafer at 1,000 r.p.m. for 30 s, followed by 1-μm thick photoresist (SU8-2001) at 3,000 r.p.m. for 30 s. After baking the photoresist at 95 °C for 1 min, ultraviolet light is exposed through a Chrome mask using a 5X stepper (GCA Autostep 6300 i-line). After developing the photoresist, the wafer is exposed to O 2 plasma for 2 min to remove the sacrificial layer. A 150-nm nickel layer is then evaporatively deposited onto the photoresist, followed by a 10-nm gold layer. The wafer is then soaked in 1H,1H,2H,2H-perfluorooctanethiol (Sigma) for 8 h to promote the formation of a self-assembled monolayer on the gold surface. Finally, gentle sonication in water releases the microbuttons by dissolving the sacrificial layer. Electromagnet and microbutton magnetic moment calibration We used a Hall probe to directly measure the magnetic field established by two independently controlled pairs of electromagnets, and measured the frequency- and amplitude dependence of both the current in the coils and the magnetic field. To determine the magnetic moment of the microbuttons, we measured their dynamic response in liquids of known viscosity. Placing the microbutton at a clean, surfactant-free air/water interface ( Bo =1), we measured the microbutton orientation under an applied, oscillatory magnetic field. As ζ r =4 πηa 3 in the low-Bo (surfactant-free) limit, we extracted the magnetic moment from measured rotational resistance via m = ωθ 0 / B 0 ζ r . In this manner, we measured the magnetic moments of 29 individual microbuttons, each with 150-nm Ni and 10-nm Au layers, from two different synthesis batches, and found m =(4.0±0.7)×10 −10 e.m.u. General experiment procedure DPPC domain structures are visualized by adding 0.1 mol% of Texas red 1,2-dihexadecanoyl- sn -glycero-3-phosphoethanolamine (DHPE, Invitrogen) to DPPC (Avanti Polar Lipids) in chloroform, which is excluded from the LC domains [2] , [35] so that disordered, LE phases appear bright in the images. A Teflon Langmuir trough is cleaned with acetone, isopropanol and deionized water at least three times. The Langmuir trough is filled with deionized water (Milli-Q). DPPC/DHPE solution is then spread at the air/water interface with micro-syringe. Chloroform evaporates to leave a surfactant monolayer. A few drops of microbuttons in deionized water are added to the trough, centred between the electromagnets. The microbuttons do not 'see' the interface, and sink. The monolayer is compressed to the LC/LE coexistence phase ( ∼ 6 mN m −1 ), and a rare earth magnet is then used to pull the microbuttons from the bottom of the trough to the air/water interface, where their amphiphilic nature 'pins' them. The monolayer is then further compressed until the desired pressure, with the rigidity of the LC/LE interface preventing microbuttons from drifting out of the field of view during compression. Two pairs of independently controlled electromagnets are used to exert a specified torque on the microbutton probe, and its resulting rotation is measured in real time by accurately locating the centroids of the buttonholes [36] . By exerting a known torque τ 0 e iωt and measuring the resulting angular displacement θ 0 e i(ωt+δ ) , we extract the rotational drag coefficient ζ r ( ω ) from the relation i ωζ r ( ω ) θ 0 e i(ωt+δ ) = τ 0 e iωt . Relating rotational drag to rheological properties Having measured the rotational drag coefficient of the microbutton probe, ζ r ( ω ), we use hydrodynamic theory to extract the viscoelastic moduli that give rise to this drag. The resistance ζ r ( ω ) is generally complex and frequency dependent, and depends on the visco(elastic) moduli of the surface and bulk phases. Just as the Stokes flow around a translating sphere must be solved to determine the steady drag of a small sphere ( F D =6 πηaU ), the Stokes flow around a rotating disc in a surfactant monolayer must be solved [37] , [38] to relate ζ r ( ω ) to surface complex viscosity η s *( ω ) and subphase viscosity η . The surface viscosity and elasticity are in turn related to the complex surface modulus according to . When Bo ≫ 1 (which holds in the experiments reported here), the rotational resistance becomes completely dominated by the interfacial rheology, and the subphase effectively decouples from the interface. A good approximation for the drag coefficient can therefore be obtained by solving the 2D Stokes equations, and . Symmetry requires the flow be purely in the θ -direction with no pressure gradient, giving simply ∇ r 2 u θ =0, with boundary conditions u θ =Ω a at r=a and u θ =0 as r →∞. The resulting velocity field is given by u θ =Ω a 2 / r , so that the torque on the disc is given by revealing the rotational resistance to be . How to cite this article: Choi, S.Q. et al . Active microrheology and simultaneous visualization of sheared phospholipid monolayers. Nat. Commun. 2:312 doi: 10.1038/ncomms1321 (2011).